RNA editing regulates transposon-mediated heterochromatic gene silencing Heterochromatin formation drives epigenetic mechanisms associated with silenced gene expression. Repressive heterochromatin is established through the RNA interference pathway, triggered by double-stranded RNAs (dsRNAs) that can be modified via RNA editing. However, the biological consequences of such modifications remain enigmatic. Here we show that RNA editing regulates heterochromatic gene silencing in Drosophila . We utilize the binding activity of an RNA-editing enzyme to visualize the in vivo production of a long dsRNA trigger mediated by Hoppel transposable elements. Using homologous recombination, we delete this trigger, dramatically altering heterochromatic gene silencing and chromatin architecture. Furthermore, we show that the trigger RNA is edited and that dADAR serves as a key regulator of chromatin state. Additionally, dADAR auto-editing generates a natural suppressor of gene silencing. Lastly, systemic differences in RNA editing activity generates interindividual variation in silencing state within a population. Our data reveal a global role for RNA editing in regulating gene expression. Organisms and biologists use double-stranded RNA (dsRNA) to program conserved RNA interference (RNAi) machinery, directing gene silencing through multiple molecular strategies. Endogenous small interfering RNAs (esiRNAs) derive from genomically encoded long precursor dsRNAs and have roles in post-transcriptional gene silencing [1] , [2] . Correspondingly, esiRNAs have been demonstrated to regulate diverse cellular pathways, including embryonic gene expression, viral defence and retrotransposition [3] , [4] , [5] , [6] . Interestingly, querying the esiRNA content of Argonaute (AGO) proteins reveals that germline and somatic esiRNAs are derived largely from transposable elements (TEs) and repetitive sequences, invoking a prominent role for esiRNAs as ‘guardians’ of the genome against selfish genetic elements [7] , [8] , [9] , [10] . Functionally, the roles of RNAi in the nucleus have been well characterized, particularly in fission yeast in which esiRNAs serve as an addressing system for the definition of genomic regions subjected to transcriptional gene silencing via heterochromatization [11] . In Drosophila melanogaster , position-effect variegation (PEV) has long been accepted as a reflection of heterochromatin formation, and mutations in the RNAi pathway are known modifiers of PEV [12] . The esiRNA pathway and long dsRNA precursors have similarly been implicated in heterochromatin formation in Drosophila [13] , [14] , [15] . The most concrete example of TE-mediated heterochromatin formation is perhaps the fourth chromosome in Drosophila . On this chromosome, and experimentally at other locations, PEV reporters have been shown to be strongly influenced by proximity to a Hoppel TE [16] , [17] , [18] . However, whereas the RNAi pathway has been shown to influence this system, no long dsRNA has been identified as a mechanistic silencing trigger. An alternate fate for long dsRNA occurs through the action of adenosine deaminase acting on RNA (ADAR) enzymes, which convert adenosine (A) to inosine (I) [19] . ADAR enzymes are best known for recoding A-to-I at specific sites in neuronal pre-mRNAs with complex secondary structures, a role with profound consequences for nervous system function [20] . However, ADAR enzymes can additionally modify up to 40% of adenosines in long perfectly duplex dsRNAs [21] . Indeed, deep sequencing of esiRNAs from Drosophila S2 cells indicates that a significant fraction of esiRNAs possesses adenosine to guanosine substitutions, suggesting that endogenous triggers of RNAi can serve as ADAR substrates [10] . This promiscuous activity of ADARs acts pleiotropically to destabilize dsRNA structures and thus limit siRNA efficacy, cause nuclear retention of certain target RNAs and induce Tudor-SN-mediated degradation of inosine-rich RNAs [22] , [23] , [24] . It has long been proposed that ADAR activity regulates RNAi in vivo , evidenced via genetic interactions between the two pathways and effects on transgene silencing [25] , [26] , [27] , [28] . Recent work reported that ADAR activity remodels the profile of small RNAs that occupy AGO complexes in vivo [29] . The molecular, cellular and organismal relevance of such negative regulation of the RNAi pathway by ADARs is, however, unclear. Here we show that Drosophila ADAR (dADAR) binds to and edits a long dsRNA comprising Hoppel TEs in vivo . The Hoppel dsRNAs serve as a genetic locus, triggering the silencing of related elements, including Hoppel’s own transposase. We demonstrate that dADAR functionally intersects this pathway as a general regulator of heterochromatin formation. Finally, we find that dADAR auto-editing generates a natural suppressor of RNAi, and, furthermore, that interindividual differences in dADAR activity appear to have a significant role in the modulation of silencing state between otherwise wild-type Drosophila . dADAR specifically binds to a chromosomal locus Specific ADAR modification of RNA is assumed to occur co-transcriptionally. For example, RNA editing and splicing are procedurally coupled in the mammalian ADAR2 gene, where editing creates a 3′ splice site acceptor that negatively regulates enzyme levels in vivo [30] . Indeed, the general dsRNA nature of mRNA-editing sites, which form dsRNA molecules by base pairing between intronic and coding sequences, suggests that editing and splicing must be orchestrated, and recent data indicate that most RNA editing occurs co-transcriptionally [31] . However, other studies suggest that ADAR proteins may localize to compartments independent of transcription—stored coincidentally with RNA at specific chromosomal sites or in the nucleoli [32] , [33] . To assess dADAR localization in vivo , we ectopically expressed an epitope-tagged dADAR transgene (dADAR-HA) in larval salivary glands. In addition to nucleolar staining, we observed a further site of localization in polytene nuclei ( Fig. 1a,b ). Chromosome squash preparations revealed a single intense band of dADAR-HA localization on chromosome 4 ( Fig. 1c ). To identify the genomic site of localization, we performed fluorescence in situ hybridization (FISH) for genes along the fourth chromosome, coupled with dADAR-HA protein localization. Within the limits of resolution, dADAR localized with the most distal gene on chromosome 4—the C alcium- a ctivated p rotein for s ecretion ( Caps ) locus ( Fig. 1d ). We reasoned that the Caps mRNA might be an undocumented dADAR target. Indeed, RT–PCR from Drosophila head RNA revealed a highly conserved editing site resulting in a recoding event ( Supplementary Fig. S1 ). Subsequent analyses revealed that, whereas Caps mRNAs are edited in salivary tissue when dADAR is expressed, so are transcripts of another known chromosome 4 dADAR target, dunc-13 . However, we observed no dADAR localization at the position of the dunc-13 locus ( Supplementary Fig. S2 ), undermining our assertion that dADAR was visualized at sites where single adenosines are deaminated. 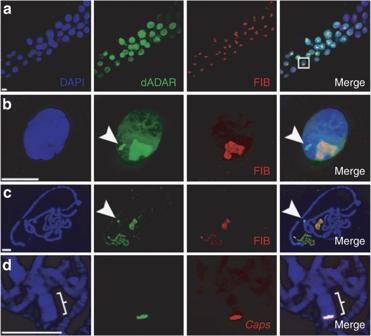Figure 1:DrosophilaADAR localizes to theCapslocus in salivary gland polytene nuclei. (a–c) Third instar larval polytene nuclei ina, magnified inband chromosomal squashes incexpressing dADAR-HA driven byelav-Gal4 and immunostained for the nucleolar marker Fibrillarin (FIB). (d) Transgenic dADAR driven byelav-Gal4 localizes to theCapslocus, labelled using a FISH DNA probe. Chromosome 4 is denoted ind. Arrows point to prominent localization of dADAR-HA on the tip of chromosome 4. Scale bars, 20 μm. Figure 1: Drosophila ADAR localizes to the Caps locus in salivary gland polytene nuclei. ( a – c ) Third instar larval polytene nuclei in a , magnified in b and chromosomal squashes in c expressing dADAR-HA driven by elav -Gal4 and immunostained for the nucleolar marker Fibrillarin (FIB). ( d ) Transgenic dADAR driven by elav -Gal4 localizes to the Caps locus, labelled using a FISH DNA probe. Chromosome 4 is denoted in d . Arrows point to prominent localization of dADAR-HA on the tip of chromosome 4. Scale bars, 20 μm. Full size image dADAR localizes to a long dsRNA source Next, we tested the sensitivity of dADAR binding on the fourth chromosome with RNAses specific to ssRNA or dsRNA ( Fig. 2a–c ). Whereas dADAR and fibrillarin proteins are removed from the nucleolus by RNAse A, a ssRNA-specific nuclease, dADAR, binding to the fourth chromosome was unchanged ( Fig. 2b ). Conversely, RNAse III, specific for dsRNA, removed detectable binding of the dADAR protein from the fourth chromosome, whereas both dADAR and fibrillarin remained localized to the nucleolus ( Fig. 2c ). 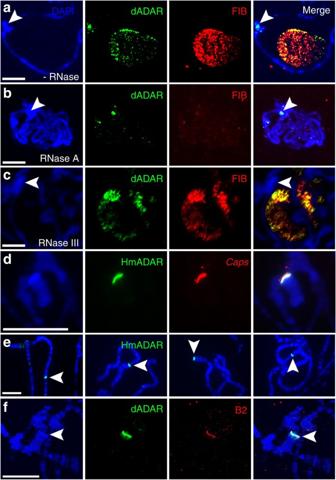Figure 2: Diverse dsRNA-binding proteins bind to a dsRNA source within theCapslocus. (a–c) Transgenic expression of dADAR-HA in polytene chromosomes not treated with RNAse ina, treated with Ribonuclease A (RNAse A) that cleaves single-stranded RNA inbor treated with Ribonuclease III (RNAse III) that cleaves dsRNA inc. (b) dADAR binding on the fourth chromosome is not abolished by RNAse A digestion (arrow). (c) RNAse III digestion results in the loss of dADAR binding on chromosome 4 (arrow) without abolishing nucleolar localization. (d) TransgenicHydra magnipapillataADAR-HA (HmADAR) driven byelav-Gal4 localizes to theCapslocus. (e) HmADAR transgene localization on a single polytene spread revealed numerous other binding locations (four examples shown) throughout the genome (arrows). (f)Elav-Gal4-driven B2-FLAG similarly localizes to theCapslocus. Arrows ina–c, andfpoint to prominent localization of dsRNA-binding proteins on the tip of chromosome 4. Scale bars, 20 μm. Figure 2: Diverse dsRNA-binding proteins bind to a dsRNA source within the Caps locus. ( a – c ) Transgenic expression of dADAR-HA in polytene chromosomes not treated with RNAse in a , treated with Ribonuclease A (RNAse A) that cleaves single-stranded RNA in b or treated with Ribonuclease III (RNAse III) that cleaves dsRNA in c . ( b ) dADAR binding on the fourth chromosome is not abolished by RNAse A digestion (arrow). ( c ) RNAse III digestion results in the loss of dADAR binding on chromosome 4 (arrow) without abolishing nucleolar localization. ( d ) Transgenic Hydra magnipapillata ADAR-HA (HmADAR) driven by elav -Gal4 localizes to the Caps locus. ( e ) HmADAR transgene localization on a single polytene spread revealed numerous other binding locations (four examples shown) throughout the genome (arrows). ( f ) Elav -Gal4-driven B2-FLAG similarly localizes to the Caps locus. Arrows in a – c , and f point to prominent localization of dsRNA-binding proteins on the tip of chromosome 4. Scale bars, 20 μm. Full size image Furthermore, we examined the localization of the epitope-tagged ADAR protein from Hydra magnipapillata (HmADAR-HA). HmADAR possesses a conserved catalytic domain and five dsRNA-binding motifs, three more than dADAR ( Supplementary Fig. S3 ). Transgenic expression of HmADAR-HA also labelled the Caps locus ( Fig. 2d ), as well as numerous additional bands throughout the genome ( Fig. 2e ). Lastly, to better understand the nature of the binding of dADAR on chromosome 4, we took advantage of the flock house virus B2 (FHV-B2) protein, which binds long dsRNA molecules in its role as a natural inhibitor of DICER cleavage and RNAi [34] , [35] . Additionally, FHV-B2 also suppresses heterochromatic gene silencing in Drosophila [15] . Co-expression of FHV-B2 and dADAR-HA proteins resulted in overlapping localization patterns ( Fig. 2f ). Furthermore, expression of the FHV-B2 protein in neurons does not alter RNA editing of the Caps transcript ( Supplementary Fig. S1f ), suggesting that FHV-B2 and dADAR do not compete for binding to the Caps mRNA-editing site. Thus far, our data are consistent with dADAR, HmADAR and FHV-B2 binding to an uncharacterized long dsRNA source near the Caps locus and further suggest that dADAR could potentially interfere with dsRNA processing and heterochromatic gene silencing in a manner analogous to FHV-B2. dADAR activity targets dsRNA generated by the Hoppel transposon Examining the architecture of the Caps locus revealed a sequence feature that could account for the abundant localization of dADAR and FHV-B2 proteins. Nested within the Caps transcription unit, we observed numerous copies of the transposable element Hoppel , three of which are tandemly repeated in an intron ( Fig. 3a,g ). Two copies are in a direct inverted repeat capable of forming an extensive (>2 kb), almost perfect dsRNA fold-back ( Supplementary Fig. S4 ). FISH for the Hoppel element revealed significant overlap with the most intense site of dADAR signal at the tip of chromosome 4 ( Fig. 3b ). In order to demonstrate that expression of the inverted Hoppel elements within Caps are sufficient for dADAR binding, we utilized mini-gene constructs containing this portion of the Caps transcription unit ( Fig. 3a ). When this mini-gene is not transcriptionally driven, no dADAR localization is detected ( Fig. 3c,d and Supplementary Fig. S5 ). In contrast, induction of mini-gene transcription with yeast Gal4 resulted in robust dADAR localization to a site ectopic to the endogenous chromosome 4 location ( Fig. 3e,f and Supplementary Fig. S6 ). 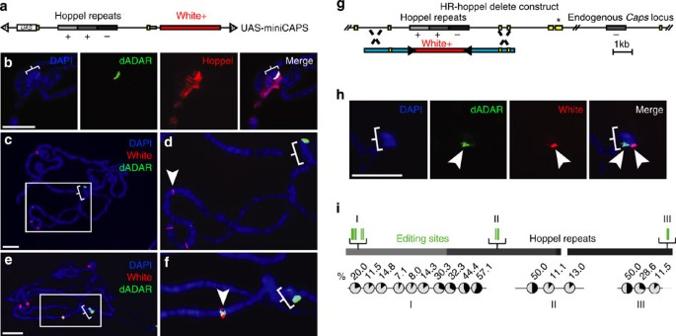Figure 3: dADAR binds to dsRNA formed by invertedHoppelelements. (a) Schematic of the UAS-miniCAPSconstruct. (b) Co-localization of dADAR andHoppelelements on chromosome 4 labelled using FISH. (c–f) dADAR does not bind to non-expressed pCasper[miniCAPS] inc, magnified indbut binds to UAS-miniCAPSdriven byelav-Gal4 ine, magnified inf. Arrows point tominiCAPSinsertions labelled via FISH formini-white+. (g) Schematic of targeting construct used to deleteHoppelelements using homologous recombination. *Edited exon ofCaps. (h) Expression of dADAR-HA in aHokmw/Hok+background. FISH formini-white+(white) indicates deleted chromatid of chromosome 4, allowing visualization of the lack of dADAR binding to theHokmwchromatid. Chromosome 4 is denoted in each image. Scale bars, 20 μm. (i) Pie charts indicating editing levels at adenosines within the threeHoppelrepeats. +/−signs inaandgdenote the orientation of transcription. Figure 3: dADAR binds to dsRNA formed by inverted Hoppel elements. ( a ) Schematic of the UAS- miniCAPS construct. ( b ) Co-localization of dADAR and Hoppel elements on chromosome 4 labelled using FISH. ( c – f ) dADAR does not bind to non-expressed pCasper[ miniCAPS ] in c , magnified in d but binds to UAS- miniCAPS driven by elav -Gal4 in e , magnified in f . Arrows point to miniCAPS insertions labelled via FISH for mini-white + . ( g ) Schematic of targeting construct used to delete Hoppel elements using homologous recombination. *Edited exon of Caps . ( h ) Expression of dADAR-HA in a Hok mw / Hok + background. FISH for mini-white + (white) indicates deleted chromatid of chromosome 4, allowing visualization of the lack of dADAR binding to the Hok mw chromatid. Chromosome 4 is denoted in each image. Scale bars, 20 μm. ( i ) Pie charts indicating editing levels at adenosines within the three Hoppel repeats. +/−signs in a and g denote the orientation of transcription. Full size image In addition to moving the Hoppel inverted repeats elsewhere, we used ends-out homologous recombination (HR) to delete three contiguous intronic repeats in Caps ( Fig. 3g and Supplementary Fig. S7 ). An intermediate of the HR process is the insertion of the mini- white + (mw) selectable eye-colour gene, which can serve as an in situ hybridization marker for the deleted chromosome. We performed in situ hybridization for white + and dADAR protein localization on heterozygotes for the Hoppel -deleted chromosome ( Fig. 3h and Supplementary Fig. S8 ). We observed robust dADAR localization on the wild-type homologue, whereas no detectable dADAR localization remained on the homologue specifically deleted for the inverted Hoppel repeats within Caps . Hoppel elements are widespread throughout the Drosophila genome. To demonstrate RNA editing of Hoppel dsRNAs arising specifically from the Caps locus, we first identified sequence polymorphisms that uniquely identified Caps -associated Hoppel elements ( Supplementary Fig. S9 ). Subsequently, we used single-molecule sequencing (SMS) to perform RNA-seq on samples of whole RNA from wild-type and dAdar null genetic backgrounds ( Fig. 3i and Supplementary Fig. S9 ). Analysis of polymorphism-containing Hoppel reads revealed that dADAR modifies multiple sites within all three transposon repeats ( Fig. 3i ). We conclude that these Hoppel inverted repeats are necessary and sufficient to generate a source of dsRNA in vivo , that dADAR and other dsRNA-binding proteins bind to this dsRNA and that dADAR deaminates multiple adenosines within this duplex RNA. Hoppel-killer ( Hok ) genetically regulates heterochromatin formation In Zea mays , the Mu-killer genetic locus ( Muk ) is an inverted repeat of the MuDR transposable element whose transcription leads to a long-hairpin dsRNA subsequently processed into siRNAs that serve to epigenetically silence mutator transposons [36] , [37] . Analogously, we propose calling the transcribed Hoppel inverted repeats within the Caps locus Hok . Our first indication that Hok could act as a genetic element triggering gene silencing came from the Hok mw deletion allele itself ( Fig. 3g ), which replaces one dose of the expressed hairpin with a copy of the mini-white gene for eye colour. Heterozygotes for this deletion ( Hok mw / Hok + ) possessing a functional copy of Hok + on the homologous chromosome show strong PEV, suggesting that the Caps region surrounding the mini-white is subjected to heterochromatic silencing, perhaps via esiRNAs generated from the Hok trigger dsRNA ( Fig. 4a,b ). These results hold for three independently targeted alleles of Hok deletions (lines Hok1 , Hok2 and Hok3 ). Cre-recombinase was used to remove the mini-white gene from Hok mw via flanking LoxP recombination sites. This deletion allele, Hok LoxP , has a single intronic LoxP site remaining. Trans-heterozygotes for both deletion alleles ( Hok mw / Hok LoxP ) still possess one mini-white reporter gene, but are fully deleted for Hok + activity, and show a strong suppression of PEV. Homozygotes for Hok mw have two doses of mini-white + and no Hok + and show maximum eye colour expression for this location ( Fig. 4a,b ). Together, these data suggest that Hok + dsRNA is capable of initiating silencing of the mini-white gene in trans . 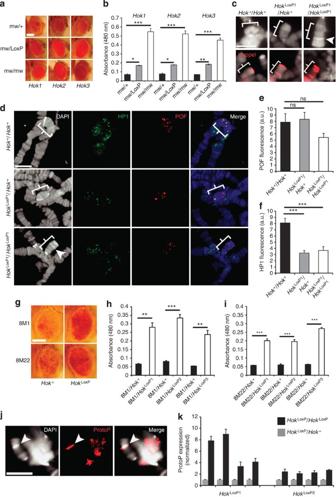Figure 4: Regulation of chromosome 4 architecture and transcription by theHoklocus. (a) Representative images of variegating and non-variegatingmini-whiteexpression in male eyes.Hok1-3indicate independentHokalleles. Scale bar, 150 μm. (b) Quantification of eye colour levels via spectral absorbance.n=3–4 independent replicates. (c) Light microscope images of chromosome 4 (upper panels) andHoppelFISH signals (lower panels). Arrow points to a prominent chromosomal band often observed inHokLoxPhomozygotes. (d) Confocal images showing HP1 and painting of the fourth (POF) localization on chromosome 4 in larvae with two (upper), one (middle) or zero (lower) copies ofHok. (e–f) Mean HP1 and POF signals normalized to DAPI intensity.n=10/genotype. (g–i) Expression of two independent chromosome 4 reporters of PEV in wild-type andHokLoxPmale eyes ing, quantified inh–iin three independentHokallelic backgrounds. Scale bar, 150 μm.n=3 independent replicates. (j) Localization ofProtoPelements on chromosome 4 and the chromocenter using a DNA FISH probe. Arrow denotes a prominent band on chromosome 4 coincident with a strongProtoPsignal. (k) The meanProtoPexpression in 2–3 day old male heads heterozygous or homozygous for two independentHokLoxPalleles.n=4 independent qPCRs. Error bars indicate s.e.m. *P<0.05, **P<0.005, ***P<0.0005; (b,e,f) one-way ANOVA with Dunnettpost-hoctest;h–i: Mann–WhitneyU-test. Scale bars inc,d, andj, 10 μm. Figure 4: Regulation of chromosome 4 architecture and transcription by the Hok locus. ( a ) Representative images of variegating and non-variegating mini-white expression in male eyes. Hok1-3 indicate independent Hok alleles. Scale bar, 150 μm. ( b ) Quantification of eye colour levels via spectral absorbance. n =3–4 independent replicates. ( c ) Light microscope images of chromosome 4 (upper panels) and Hoppel FISH signals (lower panels). Arrow points to a prominent chromosomal band often observed in Hok LoxP homozygotes. ( d ) Confocal images showing HP1 and painting of the fourth (POF) localization on chromosome 4 in larvae with two (upper), one (middle) or zero (lower) copies of Hok . ( e – f ) Mean HP1 and POF signals normalized to DAPI intensity. n =10/genotype. ( g – i ) Expression of two independent chromosome 4 reporters of PEV in wild-type and Hok LoxP male eyes in g , quantified in h – i in three independent Hok allelic backgrounds. Scale bar, 150 μm. n =3 independent replicates. ( j ) Localization of ProtoP elements on chromosome 4 and the chromocenter using a DNA FISH probe. Arrow denotes a prominent band on chromosome 4 coincident with a strong ProtoP signal. ( k ) The mean ProtoP expression in 2–3 day old male heads heterozygous or homozygous for two independent Hok LoxP alleles. n =4 independent qPCRs. Error bars indicate s.e.m. * P <0.05, ** P <0.005, *** P <0.0005; ( b , e , f ) one-way ANOVA with Dunnett post-hoc test; h – i : Mann–Whitney U- test. Scale bars in c , d , and j , 10 μm. Full size image Hoppel elements are enriched on chromosome 4 and are a target of heterochromatic gene silencing mediated by components of the RNAi machinery [16] , [17] , [18] . Given the effect on PEV, we determined the consequence of Hok deletion on the chromatin state of chromosome 4. Under ordinary light microscopy, chromosome 4 appears diffuse, non-banded and somewhat amorphous with 4',6-diamidino-2-phenylindole (DAPI) stain and is usually intimately associated with the chromocenter ( Fig. 4c ). Heterozygotes for Hok deletion somewhat maintain this appearance. However, in Hok LoxP / Hok LoxP homozygotes, chromosome 4 in its entirety appears larger in size with numerous prominent bands ( Fig. 4c and Supplementary Fig. S10 ). In addition, the chromosome 4 in situ hybridization signal for Hoppel is much more intense in Hok LoxP / Hok LoxP homozygotes compared with the wild-type or Hok LoxP / Hok + heterozygotes ( Fig. 4c ), suggesting an increased access of the Hoppel probe to chromatin. To assess molecular markers for this apparent change in the chromatin state, we performed immunohistochemistry for painting of the fourth (POF), a marker for gene activation, and heterochromatin protein 1 (HP1), a repressive mark. In keeping with the apparent change in chromosome structure, we observed a marked reduction in HP1 staining on chromosome 4, even in Hok deletion heterozygotes, without a significant decrease in painting of the fourth staining ( Fig. 4d–f and Supplementary Fig. S11 ), suggesting that loci on chromosome 4 become de-repressed in Hok mutant backgrounds. Next, we assessed the effects of Hok deletions on other silencing reporters. Two independent reporters of PEV on the fourth chromosome showed a marked decrease in PEV when placed in a heterozygous state over Hok deletion alleles, demonstrating a sensitivity to dosage of the Hok + locus, in keeping with the reduction in HP1 seen in Hok heterozygotes ( Fig. 4g–i ). One prominent band appearing on chromosome 4 in DAPI staining was observed in many preparations of Hok deletion homozygotes ( Fig. 4c,d,j ), which we hypothesized could be the site of the ProtoP transposon that is homologous to Hoppel and expresses the transposase required for mobilization of defective Hoppel elements. Indeed, hybridization probes for the ProtoP element overlap precisely with the appearance of this intense band of DAPI staining seen in Hok deletion homozygotes ( Fig. 4j ). Therefore, we quantified the somatic expression of the ProtoP transposase in Hok deletion homozygotes versus heterozygous controls and found a reproducible increase in transposase expression when Hok + dosage is reduced ( Fig. 4k ). Taken together, these data support a role for the Hok locus in serving as a trigger for heterochromatic gene silencing of chromosome 4 and indicate a regulatory role for Hok , similar to that described for Muk , in silencing an endogenous nucleic acid parasite. dADAR regulates heterochromatic state and lifespan As dADAR binds to and modifies Hok dsRNA, we assessed the genetic interaction between dADAR deficiency and silencing using reporters of PEV in a defined dAdar null allele ( dAdar 0 ) ( Supplementary Fig. S12 ). For two independent alleles of Hok mw that variegate and two other chromosome 4 reporters of PEV, dADAR deficiency strongly enhanced PEV ( Fig. 5a,b and Supplementary Fig. S13 ), suggesting that dADAR normally acts to oppose silencing on chromosome 4, through Hok + dsRNA. To assess whether this reflects more global changes, we measured levels of HP1, the silencing histone marks H3K9 (monomethyl and dimethyl) and the histone activation mark H3K4 (trimethyl) in wild-type and dAdar 0 Drosophila heads. We saw no change in HP1 levels in response to changing dADAR levels. However, we saw opposing effects on histone silencing and activation marks in response to dADAR deficiency ( Fig. 5c,d ), indicating that the loss of dADAR activity leads to a significant increase in global silencing within the nervous system. In keeping with these changes seen in whole-head extracts, we observed a significant increase in the extent of nuclear H3K9me2 staining in whole mount adult dAdar 0 Drosophila neurons compared with wild-type controls ( Fig. 5e–j and Supplementary Fig. S14 ). Consistent with western blot results, we observed no change in HP1 levels. 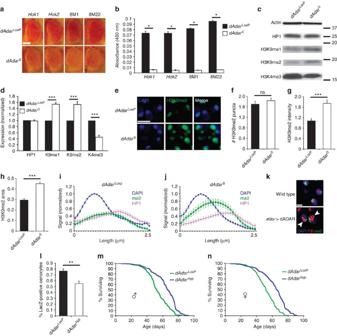Figure 5: RNA editing regulates heterochromatic gene silencing. (a) Representative images of control (dAdarLoxP) ordAdarnull (dAdar0) male eyes expressingmini-whitereporters of PEV located on chromosome 4, including two independentHokmwalleles. Scale bar, 150 μm. (b) The mean pigmentation levels of the four reporters in control anddAdar0eyes.n=4 independent replicates. (c) Western blots of silencing and activating chromatin marks in control anddAdar0head samples. (d) Quantification of HP1 and histone methylation levels, normalized to Actin.n=7–12 western blots. (e) Confocal slices showing dimethyl H3K9 (H3K9me2) expression in control anddAdar0adult neuronal nuclei. Scale bar, 5 μm. (f–h) Properties of H3K9me2 puncta in control anddAdar0adult neuronal nuclei.n=30 nuclei/genotype. (i–j) Average linear signal intensities for DAPI, H3K9me2 and HP1 immunostaining across the neuronal nuclei in control (n=25 nuclei) anddAdar0(n=20) adult brains (see Methods for details). Values were normalized to the peak DAPI signal. (k) Salivary gland nuclei labelled with antibodies against FIB and H3K9me2 (me2). Note the irregular nucleolar morphology in nuclei overexpressing dADAR (arrows, lower panel) relative to controls (upper panel). Scale bar, 20 μm. (l) Expression of a Lac-Z-based reporter of gene silencing (see Methods) in control (dAdarLoxP) anddAdarhypoenocytes.n=30/genotype. (m–n) Lifespan curves for wild-type anddAdarhypmales inmand females inn(seeSupplementary Table S1forn-values and statistics). Error bars indicate s.e.m. *P<0.05, **P<0.005, ***P<0.0005, Mann–WhitneyU-test. Figure 5: RNA editing regulates heterochromatic gene silencing. ( a ) Representative images of control ( dAdar LoxP ) or dAdar null ( dAdar 0 ) male eyes expressing mini-white reporters of PEV located on chromosome 4, including two independent Hok mw alleles. Scale bar, 150 μm. ( b ) The mean pigmentation levels of the four reporters in control and dAdar 0 eyes. n =4 independent replicates. ( c ) Western blots of silencing and activating chromatin marks in control and dAdar 0 head samples. ( d ) Quantification of HP1 and histone methylation levels, normalized to Actin. n =7–12 western blots. ( e ) Confocal slices showing dimethyl H3K9 (H3K9me2) expression in control and dAdar 0 adult neuronal nuclei. Scale bar, 5 μm. ( f – h ) Properties of H3K9me2 puncta in control and dAdar 0 adult neuronal nuclei. n =30 nuclei/genotype. ( i – j ) Average linear signal intensities for DAPI, H3K9me2 and HP1 immunostaining across the neuronal nuclei in control ( n =25 nuclei) and dAdar 0 ( n =20) adult brains (see Methods for details). Values were normalized to the peak DAPI signal. ( k ) Salivary gland nuclei labelled with antibodies against FIB and H3K9me2 (me2). Note the irregular nucleolar morphology in nuclei overexpressing dADAR (arrows, lower panel) relative to controls (upper panel). Scale bar, 20 μm. ( l ) Expression of a Lac-Z-based reporter of gene silencing (see Methods) in control ( dAdar LoxP ) and dAdar hyp oenocytes. n =30/genotype. ( m – n ) Lifespan curves for wild-type and dAdar hyp males in m and females in n (see Supplementary Table S1 for n -values and statistics). Error bars indicate s.e.m. * P <0.05, ** P <0.005, *** P <0.0005, Mann–Whitney U- test. Full size image Does dADAR modulate other measures of heterochromatin state, namely, transposon transcription level and nuclear morphology? We found that the loss of dADAR resulted in a marked increase in silencing for three out of five transposable elements tested ( Supplementary Fig. S15 ), as expected if dADAR activity opposes silencing via the RNAi pathway for particular classes of transposon. Differential effects of RNAi mutants (for example, Ago2) on repeat expression, as well as ADAR’s selective influence on particular dsRNA trigger loci, have been reported previously [7] , [29] . If the effects we observe are mediated by the binding of dADAR to dsRNA intermediates, we reasoned that overexpression of dADAR, and potentially other dsRNA-binding proteins, might mimic loss-of-function mutations in the RNAi pathway. Fragmentation of the nucleoli and derangement of the normal pattern of silencing marks associated with heterochromatin within the nucleus has been previously observed in RNAi mutants [38] . Similarly, we found that the overexpression of dADAR, HmADAR or FHV-B2 proteins in salivary glands led to nucleolar fragmentation and a delocalization of H3K9me2 staining in the nuclei ( Fig. 5k and Supplementary Fig. S16 ). As complete loss of dADAR protein increases silencing levels, we assessed whether altering the dosage of dADAR also had measurable effects. Reduction of dADAR by 50% in dAdar 0 /+ heterozygous females increased silencing of four PEV reporters ( Supplementary Fig. S17 ). Previously, we described a hypomorphic allele of dAdar ( dAdar hyp ) that results in an ~80% reduction in dADAR levels and a concomitant decrease in specific editing [39] . We tested the effect of dAdar hyp on a previously characterized lacZ PEV reporter expressed in Drosophila oenocytes [40] . The expression of this reporter was reduced in a dAdar hyp background ( Fig. 5l ), indicative of increased silencing. As a loss of silencing has been associated with aging in Drosophila and other organisms [41] , [42] , we performed lifespan analyses on dAdar hyp adults and wild-type controls and found an ~20% increase in the median lifespan in dAdar hyp males and females ( Fig. 5m,n and Supplementary Table S1 ). Thus, reporters of gene silencing, chromatin modifications and organismal phenotypes all respond in a direction consistent with dADAR activity having a role in the regulation of heterochromatic gene silencing by antagonizing the endogenous RNAi pathway. dADAR auto-editing generates a suppressor of gene silencing We previously reported that dADAR auto-editing produces a serine (S) to glycine (G) change in the catalytic domain of dADAR that acts to negatively tune dADAR activity [43] . In addition, the edited (G) version of dADAR localized to a novel intranuclear punctus, suggesting an unknown role for RNA editing in the nucleus. We assessed the effect of these two versions of dADAR using genetically engineered alleles that produce equal amounts of the unedited or edited protein isoforms, dADAR S and dADAR G , respectively. Paradoxically, we found that auto-editing (dADAR G ) profoundly suppresses PEV of four reporters compared with the editing-competent wild-type allele (dADAR LoxP ; Fig. 6a–e ). The allele that produces only unedited dADAR (dADAR S ) showed an enhancement of PEV compared with the control. Similarly to dAdar hyp , dAdar S animals exhibit an increase in the median lifespan ( Supplementary Fig. S18 and Supplementary Table S1 ), consistent with the notion that increased silencing extends lifespan. We then assessed HP1 levels in brain tissue of these mutants and found a substantial reduction in HP1 levels in dADAR G -expressing neurons ( Fig. 6f–h and Supplementary Fig. S13 ), indicative of a loss in silencing. Thus, in contrast to its modest reduction of deaminase activity on specific mRNA targets, dADAR G appears to have a strong dominant and suppressive effect on gene silencing. 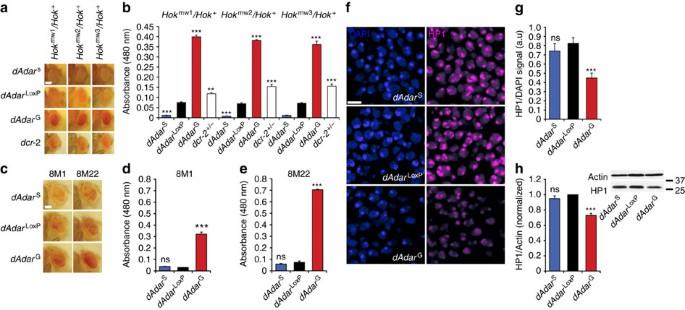Figure 6: dADAR auto-editing generates a suppressor of gene silencing. (a,b) AlteredHokmwexpression in males with bidirectional modifications indAdarauto-editing and indcr-2mutants (examples shown inaquantified inb). Scale bar, 150 μm.n=4 independent samples. (c–e) Independent PEV reporter expression indAdarauto-editing mutants.n=5 independent samples. Scale bar, 150 μm. (f) Confocal slices showing HP1 expression in the neuronal nuclei from control anddAdarauto-editing mutant adult male brains. Scale bar, 5 μm. (g) Mean HP1 levels in control and auto-editing mutant nuclei, normalized to the DAPI signal.n=22–25 nuclei/genotype. (h) Representative western blots (inset) and quantification of HP1 protein levels in control and auto-editing mutant head samples. Values were normalized to Actin-loading controls. Mutant HP1 levels are normalized todAdarLoxpcontrols.n=8 independent western blots. Error bars indicate s.e.m. *P<0.05, **P<0.005, ***P<0.0005, one-way ANOVA with Dunnettpost-hoctest. Figure 6: dADAR auto-editing generates a suppressor of gene silencing. ( a , b ) Altered Hok mw expression in males with bidirectional modifications in dAdar auto-editing and in dcr-2 mutants (examples shown in a quantified in b ). Scale bar, 150 μm. n =4 independent samples. ( c – e ) Independent PEV reporter expression in dAdar auto-editing mutants. n =5 independent samples. Scale bar, 150 μm. ( f ) Confocal slices showing HP1 expression in the neuronal nuclei from control and dAdar auto-editing mutant adult male brains. Scale bar, 5 μm. ( g ) Mean HP1 levels in control and auto-editing mutant nuclei, normalized to the DAPI signal. n =22–25 nuclei/genotype. ( h ) Representative western blots (inset) and quantification of HP1 protein levels in control and auto-editing mutant head samples. Values were normalized to Actin-loading controls. Mutant HP1 levels are normalized to dAdar Loxp controls. n =8 independent western blots. Error bars indicate s.e.m. * P <0.05, ** P <0.005, *** P <0.0005, one-way ANOVA with Dunnett post-hoc test. Full size image Interindividual variation in ADAR affects gene silencing PEV reporter lines display a range of expression of the variegating phenotype within their population. We previously reported interindividual differences in dADAR activity using an editing-dependent reporter construct [44] . Given that both dADAR levels and auto-editing states strongly affect silencing, we were curious to determine the degree to which variation in PEV might be attributed to interindividual dADAR levels, which would directly determine the absolute amount of dADAR G produced. We classified PEV phenotypes in wild-type and dAdar mutant populations into three distinct groupings based on eye colour: almost no eye pigment (category 1, indicative of strong silencing), almost wild-type eye colour (category 3, indicative of weak silencing) and intermediate phenotypes (category 2, PEV) ( Fig. 7a ). The auto-editing status clearly modulated the abundance of the three classes of PEV ( Fig. 7a ). Hard-wiring auto-editing (dADAR G ) results in an almost complete shift to category 3, whereas dADAR S results in all category 1. We next isolated animals from the dADAR LoxP wild-type control that represented the extremes of PEV eye expression range—categories 1 and 3. We then assessed the level of specific editing in thorax tissue of these animals for 30 dADAR target adenosines and present the results as the mean editing level of category 3 normalized to category 1. We observed that for the majority of sites, editing levels were higher for category 3 (decreased silencing) compared with category 1 (increased silencing) ( Fig. 7b and Supplementary Table S2 ). These results are consistent, with higher dADAR levels being present systemically in category 3 individuals compared with category 1 animals. Therefore, we propose that a substantial amount of the variability in phenotype within populations containing PEV reporters (an indirect measure of chromatin silencing) could arise from whole animal, interindividual differences, in dADAR levels or activity acting through the function of dADAR G as an inhibitor of RNAi-mediated silencing. 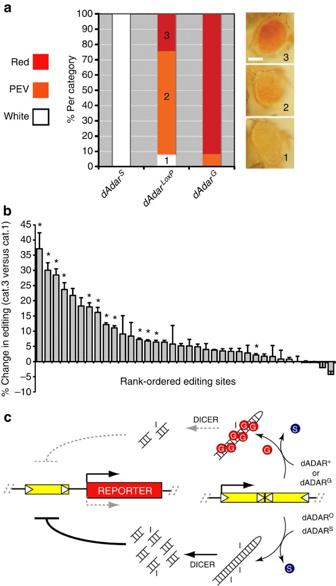Figure 7: Interindividual variation in heterochromatic gene silencing through ADAR activity. (a) Representative examples (right) and percentages of categories ofHokmw/Hok+PEV reporter expression observed in wild-type anddAdarauto-editing mutant backgrounds, ndAdarS=572, ndAdarLoxp=492 and ndAdarG=534. Scale bar, 150 μm. (b) Editing levels at 30 dADAR target adenosines, presented as the % editing in category 3 thorax tissue normalized to the mean editing in category 1 thorax tissue for each site. (c) Speculative model of the functional consequences of dADAR auto-editing on PEV reporter expression via differential modulation of the small RNA pathway. Error bars indicate s.e.m. *P<0.05, **P<0.005, ***P<0.0005, Mann–WhitneyU-test. Figure 7: Interindividual variation in heterochromatic gene silencing through ADAR activity. ( a ) Representative examples (right) and percentages of categories of Hok mw /Hok + PEV reporter expression observed in wild-type and dAdar auto-editing mutant backgrounds, n dAdar S =572, n dAdar Loxp =492 and n dAdar G =534. Scale bar, 150 μm. ( b ) Editing levels at 30 dADAR target adenosines, presented as the % editing in category 3 thorax tissue normalized to the mean editing in category 1 thorax tissue for each site. ( c ) Speculative model of the functional consequences of dADAR auto-editing on PEV reporter expression via differential modulation of the small RNA pathway. Error bars indicate s.e.m. * P <0.05, ** P <0.005, *** P <0.0005, Mann–Whitney U- test. Full size image We pursued an observation of the in vivo localization of the RNA-editing enzyme, dADAR, to the proof of its action on an endogenously expressed inverted repeat of the TE, Hoppel . Our results explicitly demonstrate a functional intersection between the processes of RNA editing and RNA silencing. Previous studies in Drosophila implicate Hoppel and the RNAi pathway in determining the global silencing state of chromosome 4, although no dsRNA trigger had been experimentally identified [13] , [14] . We show that the inverted repeat acts as a genetic element, Hok , and regulates PEV, the global architecture of chromosome 4, and silences the Hoppel transposase. As a general mechanism, ADAR's action on dsRNA should oppose RNAi. We show that deficiency for ADAR acts as a global enhancer of silencing state, and dADAR hypomorphism even extends lifespan. In Drosophila , gene silencing decreases with age and has been implicated in the aging process [41] . Thus, substantial decreases in ADAR activity may lead to lifespan extension through increased silencing. Interestingly, polymorphisms within a human ADAR gene have been associated with extreme longevity, indicating that interventions involving ADAR activity may be capable of affecting lifespan [45] . Importantly, mutations in human ADAR1 cause Aicardi–Goutières syndrome in which it is hypothesized that ADAR has a role in regulating dsRNA metabolism from repeated elements in the human genome [46] . Thus, our data are consistent with a conserved role in the regulation of dsRNA levels in animals through RNA editing or RNA binding. Mechanistically, we provide evidence that dADAR auto-editing has evolved as a natural inhibitor of RNAi, generating dADAR G . In dAdar null or dAdar S genetic backgrounds, no dADAR G can be produced. Thus, both backgrounds effectively act as enhancers of PEV (E(var)). In the wild-type background, PEV occurs to the extent that each animal expresses dADAR (and the corresponding amount of dADAR G ). In the extreme, the dAdar G background acts as a strong suppressor of PEV (Su(var)). How can a single amino acid change in dADAR protein affect such a silencing switch? We speculate that dADAR G may interfere indirectly with Dicer activity on dsRNA, simply by blocking access via binding irrespective of editing activity, analogous to the FHV-B2 protein ( Fig. 7c ). Alternately, a recent study showed a direct functional interaction between mammalian ADAR and Dicer that is necessary for the processing of small RNAs [47] . If dADAR has a similar interaction, it could also mediate all of the effects in our model ( Fig. 7c ) via dominant-negative interactions of dADAR G with Dicer, whereas dADAR S (which encodes the conserved amino acid) would function in a similar manner described in mammals to promote small RNA biogenesis. Further biochemical experiments will be necessary to determine whether this phenomenon is conserved across species and the exact molecular mechanisms through which dADAR G exerts its effects. The most engaging aspect of our results lay in their implications for somatic regulation of heterochromatin functioning as a safeguard of transposon activity, especially in the nervous system. The RNA-induced silencing complex isolated from Drosophila tissue-culture cells was shown to be programmed with esiRNAs, largely derived from transposon sequences, a significant portion of which bears the signature of a single dADAR modification [10] . Likewise, in C. elegans , ADAR activity has a profound effect on the abundance and identity of small RNA profiles [29] . Further experiments in this system using deep sequencing technologies will be necessary to shed light on the effects of ADAR on endo-siRNA abundances and functionality. We envision that such RNA-editing-mediated effects may be quite specific to the nature of individual dsRNA triggers. Studies in both mammals and Drosophila have shown that TEs are mobile in the nervous system, revealing an intriguing mechanism for the generation of somatic mutations potentially conferring adaptive value in individuals [48] , [49] , [50] . Here we demonstrate a mechanistic link between RNA editing and the regulation of transposon silencing, particularly in the nervous system, which may have domesticated uses as diversifiers of neuronal genomes on a neuron-to-neuron and an individual-to-individual basis. The implications of our results, given the universal prevalence of dsRNAs as a component of transcriptomes, are that ADAR activity has an evolved role in determining the fate of RNAs entering silencing pathways, thus globally influencing somatic genomic integrity, gene expression and downstream organismal phenotypes. Drosophila stocks and HR Drosophila strains were raised at a constant 25 °C, on standard molasses food, and under 12 h day/night cycles. Tissue-specific Gal4 lines were obtained from the Bloomington stock center. Stocks of D. simulans, D. sechellia, D. yakuba and D. erecta were obtained from the Drosophila Species Stock Center (University of California, San Diego). We performed ends-out HR using a similar methodology to that reported previously [51] .Briefly, we utilized the ends-out targeting vector p[w25.2] that contains the white+ selectable eye colour mini-gene flanked by LoxP sites for subsequent removal by Cre-recombinase. Homology arms were cloned and sequenced in pTOPO (Invitrogen) and then shuttled into the multiple cloning sites of the vector to generate the Hoppel deletion alleles, which were then introduced into the Drosophila genome using standard transgenic methods (Genetic Services Inc.). The cloning strategy is as follows: where all genomic coordinates are given by the D. melanogaster draft, BDGP Release 5, with release 5.12 annotation provided by FlyBase at the UCSC Genome Browser. Arm 1 is the 5′ arm of p[w25- Hok ] and was generated using PCR amplification to incorporate cloning sites as follows: Arm 1, Bsi WI-1,258,227–1,260,758- Asc I. Arm 2, is the 3′ arm of p[w25- Hok ] and was generated using PCR amplification to incorporate cloning as follows: Arm 2, Acc 65I-1,264,090–1,266,567- Not I. Targeting was performed to generate multiple independent targeting Hok alleles. Targeted alleles were validated by amplification using primers outside the region of targeting ( Supplementary Fig. S7 ). Subsequent removal of the white mini-gene selectable marker was achieved by performing crosses to animals expressing Cre-recombinase and re-isolation of targeted chromosomes containing a single LoxP site. The recombinant alleles were subsequently back-crossed to WT background for five generations. Microscopy and immunohistochemistry All confocal images were obtained on a Zeiss LSM 510 meta confocal microscope. Adult brain and third instar larval salivary glands were fixed in 4% paraformaldehyde (PFA) and blocked in 5% normal goat serum before antibody incubation. Primary antibodies were used at the following concentrations: rabbit anti-HA (Santa Cruz Biotechnology), 1:50; goat anti-human fibrillarin (kind gift of K.M. Pollard, TSRI, San Diego, CA, USA), 1:200; anti-HP1 antibody (Developmental Studies Hybridoma Bank (DSHB), C1A9; 1:100); H3K9me2 (kind gift of T. Jenuwein; 1:100) DAPI (Invitrogen) was used at 1:1,000. Images were contrast-enhanced in Adobe Photoshop. Polytene squashes were imaged using either confocal microscopy or epifluorescence. A Zeiss AX10 Imager.M1 was used for epifluorescence imaging. Alexa Fluor-conjugated secondary antibodies (goat anti-mouse Cy3, goat anti-rabbit 488 and goat anti-rabbit Cy5 (Invitrogen Molecular Probes)) were used at 1:200. Third instar larval salivary glands were dissected in 45% acetic acid and transferred to a fixative solution for 3–5 min. The salivary gland nuclei were squashed for spreading of the polytene chromosomes on a siliconized slide. Each slide was immersed in liquid nitrogen and washed in room temperature in EtOH (5 min), in 1 × PBST twice (10 min) and in phosphate-buffered saline (PBS) (10 min). The chromosomes were placed in a blocking solution (PBS: 0.5% bovine serum albumin) for 30 min prior to immunohistochemistry [52] . To examine the distribution of the H3K9me2 and HP1 signals relative to DAPI in adult Drosophila neuronal nuclei ( Fig. 5 ), a linear region of interest was drawn for each cell beginning before the peak area of DAPI signal and placed to incorporate the foci of H3K9me2 and HP1 within the nucleus. The peak DAPI signal was set to an arbitrary value of 1 and the remaining DAPI, H3K9me2 and HP1 signals were normalized to this value. In both dAdar Loxp and dAdar 0 brain nuclei, DAPI signals exhibited a foci of relatively high DAPI levels. Both H3K9me2 and HP1 also exhibited nonuniform patterns of distribution. In some cells, foci of both signals were closely associated with increased DAPI signals; however, in others the silencing mark foci were non-overlapping with the DAPI foci. However, the mean peak of the H3K9me2 signal, but not the HP1 signal, was clearly higher in dAdar 0 brain nuclei relative to dAdar Loxp . Western blotting Whole-head lysates were prepared from 30-adult male heads per 100 μl of RIPA buffer (150 mM NaCl, 1.0% NP-40, 0.5% Sodium Deoxycholate, 0.1% SDS, 50 mM Tris-HCl pH8.0), including 1 mM DTT, 1 mM PMSF and protease inhibitor mixed tablet (Roche). Approximately 25 μg per sample were mixed in 6 × sample buffer containing SDS and β-mercaptoethanol and loaded on 12.5% SDS–PAGE gels and then transferred on 0.2-um-pore size polyvinylidene difluoride membranes (Bio-Rad). The primary antibodies were anti-actin antibody (Millipore, C4; 1:40,000), anti-HP1 antibody (DSHB, C1A9; 1:750), H3K9me (T. Jenuwein; 1:2,000), H3K9me2 (T. Jenuwein; 4,858; 1:1,000–1,500) and H3K4me3 (Abcam, ab8580; 1:1,500). Secondary antibodies were as follows: HRP-conjugated goat anti-mouse (Abcam; 1:6,000–10,000) and goat anti-rabbit (Bio-Rad). Band intensities of histone marks were quantified on ImageJ following background subtraction. RNA-editing analysis To analyse RNA-editing levels, total RNA was extracted from heads (20 per sample) of 1- to 2-day-old male Drosophila . RNA extractions were performed using TRIzol reagent (Invitrogen). Edited cDNAs were amplified via RT–PCR using target-specific primers for known dADAR target transcripts as described previously [43] . Levels of RNA editing were calculated by measuring the area under A and G peaks in individual electropherogram traces using ImageJ. The per cent editing is expressed at G/(A+G) × 100. To analyse editing in flies exhibiting differing degrees of PEV, total RNA was isolated from male Drosophila thoraxes (20 per sample). A minimum of three independent PCR amplicons were used to derive the extent of RNA editing. Eye-pigmentation and LacZ PEV assays For eye pigmentation assays, flies were raised at 25 °C. Heads of 40 male or female flies (2–3 days old) of each genotype were placed in methanol and acidified with 0.1% HCl at 4 °C overnight for pigment extraction. Heads were homogenized and eye pigmentation was represented as the absorbance of the supernatant at 480 nm. For LacZ PEV assays, flies were housed in a humidified, temperature-controlled incubator under 12 h day/night cycles at a constant 25 °C. Flies were aged on food containing 12% sucrose, 3% yeast and 5% corn until 30 days of age. Virgin dAdar hyp and dAdar LoxP homozygote female flies were crossed with male BL2 flies containing the HS- LacZ construct as described previously [53] . At 30 days, male progeny flies ( dAdar hyp , dAdar LoxP ) were heat-shocked at 37 °C for 40 min and allowed to recover at 25 °C for 40 min. Small holes were punched in the exoskeleton. Flies were fixed in 4% paraformaldehyde for 10 min, washed in PBS and then stained in staining solution containing 0.25% X-gal at room temperature overnight. Abdomens were dissected in order to visualize oenocyte cells, and the total number of both stained and unstained oenocytes was recorded. The percentage of stained oenocytes was determined for 30 individual flies per genotype. FISH and RNAse treatment FISH probes were generated from PCR products using the following primers: Caps F-5′-CTGTTGATTATATAGAAGCCGCCAGTG-3′, Caps R-5′-CACCTTGAATTTTCGACATAGCTGAGTT-3′, white F-5′-GGAGCAGCCGGAGAATGGGTAC-3′, white R-5′-GCTCCAGCTCCTCGACCGCGTCC-3′, Hoppel F-5′-GGCCGTGGCTCTAGAGGTGGATCCA-3′, Hoppel R-5′-GCGTAACTGCCATACATTAGTTTGGC-3′, ProtoP F-5′-GTTCGATTCGATAATATATCAGCC-3′, ProtoP R-5′-CTATATTTTGGTCAAAGTACCTCTC-3′. Probes were labelled directly with biotine-16-dUTP (Roche). Larvae were dissected in 45% acetic acid and transferred to a fixative solution for 5 min. Slides were frozen in liquid nitrogen and washed in ethanol and PBS for 10 min each. The chromosomes were placed at 70 °C in 2 × SSC for 45 min. The chromosomal DNA was denatured in 0.14 M NaOH/2 × SSC for 3 min and subsequently washed in 70% ethanol for 20 min and 95% ethanol for 10 min. The FISH probe was hybridized to the polytene chromosomes at 37 °C for 20 h. An anti-biotin Texas Red secondary antibody (Abcam) was used to detect the FISH probe. RNAse treatment of polytene chromosomes with RNAse A (New England Biolabs) and RNAse III (New England Biolabs) was carried out according to the manufacturer’s instructions. Briefly, salivary glands were dissected at room temperature and incubated with RNAse A and RNAse III for 10 min. Salivary glands were then transferred for fixation in a formaldehyde solution for 15 min. Quantitative RT–PCR analysis For quantitative RT–PCR analysis of transposable elements and ProtoP transposase, total RNA (5 μg) was extracted from heads (50 per sample) of 1- to 2-day-old male Drosophila from each genotype tested. Total RNA was extracted using TRIzol reagent (Invitrogen), treated with DNase I (Ambion), and reverse transcribed using the Bio-Rad iScript cDNA synthesis kit according to the manufacturer’s instructions. cDNA (50 ng) was then analysed in quadruplicate via quantitative RT–PCR in a 7,500 fast real-time PCR machine using the SYBR green PCR master mix. Relative RNA levels were determined from the threshold cycle for amplification, and GAPDH was used as an internal control. The primers used in this study for DM297, Gypsy6, BEL1 and F-element transposable elements expression were described previously [7] . The primers used for the 1,360 transposable element expression have also been described previously [17] .Primers used for expression analysis of GAPDH and ProtoP are as follows: F-5′-GACGAAATCAAGGCTAAGGTCG-3′, R-5′-AATGGGTGTCGCTGAAGAAGTC-3′ and F-5′-GTATGATCAAGGAGGTAACAATAG-3′, R-5′-CCTTACAGACTTGAAAAGATGCGG-3′, respectively. Single-molecule sequencing We used the SMS RNAseq data set described in (Sequence Read Archive accession number SRP028559 ) [54] . Briefly, total RNA from whole Canton-S (WT) and dAdar 5g1 flies was isolated using TRIzol reagent (Invitrogen) following the manufacturer’s protocol and treated with TurboDNase (Ambion). The RNA was then depleted of rRNA using the RiboMinus Eukaryote kit (Invitrogen) and converted to single-stranded cDNA using random-hexamers with the Superscript III kit (Invitrogen). The cDNA was then polyA-tailed and 3′-blocked using terminal transferase and sequenced on a Heliscope [54] . The SMS reads were aligned to Drosophila genomic sequence DM3 supplemented with all possible splice junctions as described in Laurent et al . [54] with the exception that the read uniqueness filer was turned off allowing for mapping of reads in repetitive regions. Then, we selected SMS reads that could be unambiguously assigned to the Hoppel repeat located in the Caps locus based on the presence of the unique polymorphisms as described in the legend to the Supplementary Fig. S9 These reads were then passed through in-house editing site discovery pipeline developed previously by us for unbiased whole-genome detection of RNA-editing sites in Drosophila [54] . Briefly, the pipeline consisted of successive application of a number of filters to remove sequencing and biological artifacts. The filters were calibrated based on iterative process in which result from each iteration was tested by Sanger-based validation of a random subset of sites. After each iteration, the filters were adjusted to increase the validation rates. The final validation rate of our set of whole-genome editing sites was ~87% (ref. 54 ). Lifespan and fertility assays All lifespan and fertility experiments were performed in a humidified, temperature-controlled incubator under 12-h day/night cycles at a constant 25 °C. Flies were collected under light anaesthesia and housed at a density of 25 males and 25 females each per vial. Flies were passed every day and the number of dead flies was recorded. All lifespan experiments were performed on food containing 15% yeast and 15% sucrose without added live yeast. For fertility assays, flies were collected under light anaesthesia and housed at a density of one male and two females each per vial. Flies were passed every day and the number of eggs recorded for 20 days. All fertility experiments were performed on food containing 15% yeast and 15% sucrose without added live yeast. How to cite this article: Savva, Y. A. et al . RNA editing regulates transposon-mediated heterochromatic gene silencing. Nat. Commun. 4:2745 doi: 10.1038/ncomms3745 (2013).